Antagonistic roles ofDrosophilaTctp and Brahma in chromatin remodelling and stabilizing repeated sequences Genome stability is essential for all organisms. Translationally controlled tumour protein (TCTP) is a conserved protein associated with cancers. TCTP is involved in multiple intracellular functions, but its role in transcription and genome stability is poorly understood. Here, we demonstrate new functions of Drosophila TCTP (Tctp) in transcription and the stability of repeated sequences (rDNA and pericentromeric heterochromatin). Tctp binds Brahma (Brm) chromatin remodeler to negatively modulate its activity. Tctp mutants show abnormally high levels of transcription in a large set of genes and transposons. These defects are ameliorated by brm mutations. Furthermore, Tctp promotes the stability of repeated sequences by opposing the Brm function. Additional regulation of pericentromeric heterochromatin by Tctp is mediated by su(var)3-9 transcriptional regulation. Altogether, Tctp regulates transcription and the stability of repeated sequences by antagonizing excess Brm activity. This study provides insights into broader nuclear TCTP functions for the maintenance of genome stability. Genome stability is critical for development and survival of all organisms. The DNA of eukaryotic genome is packaged into nucleosomes. Continuous nucleosome arrays form more complex chromatin fibers, resulting in chromosomes [1] composed of two types of domains: euchromatin and heterochromatin. In general, euchromatin is gene-rich, accessible to DNA binding factors and transcriptionally active, while heterochromatin is gene-poor [2] , [3] and transcriptionally less active [1] . However, these two domains are distinguished further by other properties, including DNA sequence composition and gene density [1] , [3] . In fission yeast, flies and mammals, pericentromeric heterochromatin is important for the regulation of sister-chromatid cohesion and centromere stability. Silencing histone marks such as H3K9me2/3, HP1a, and SU(VAR)3-9 are abundant in heterochromatin, and critical for DNA repair in highly repeated sequences [4] , [5] , homologous recombination between repetitive DNA sequences [6] , [7] and suppression of transposons [8] . Interestingly, silencing histone marks are also required for the stability and repair of rDNA sequences, which are proximal to pericentromeric heterochromatin and partially silenced in Drosophila [2] , [3] , [9] . Di/tri-methylation of histone H3K9 in heterochromatic genes and repeats is catalysed by histone SU(VAR)3-9 methyltransferase (HMT) and HP1a, which is crucial for genome stability by maintaining heterochromatin structures [6] . Besides histones, DNA packaging requires histone chaperones, histone-modifying enzymes and chromatin remodelling complexes (remodelers). Of these, chromatin remodelers are major contributors to the dynamic nature of chromatin because they use the energy from ATP-hydrolysis to organize nucleosomes [10] , [11] . These functions of remodeler complexes allow diverse proteins, such as RNA/DNA polymerases, transcription factors and DNA repair proteins, to access to the DNA and modulate transcription, DNA replication and DNA repairs. Four classes of ATPase remodelers have been identified (SWI/SNF, ISWI, CHD and INO80) according to their unique domains flanking the ATPase region: HSA and Bromo domains for SWI/SNF, SANT and SLIDE domains for ISWI, two tandemly arranged chromo domains for CHD, and HSA for INO80. In flies and mammals, mutants in these remodeler genes show various defects in development, transcription, chromatin structure formation, DNA damage repair, fertility [11] or cell proliferation [12] , [13] . The Drosophila SWI/SNF remodeler called the Brahma (Brm) complex consists of at least 11 subunits, including 7 core subunits and 4 accessories [14] , [15] . A catalytic ATPase subunit is encoded by brahma ( brm ) gene, which is essential for global transcription by RNA polymerase-II (Pol-II) [16] , inhibition of heterochromatin spreading [17] and suppression of homeotic transformation by Polycomb gene mutations [11] . There are two distinct Brm complexes in Drosophila according to their specific compositions of core and accessary subunits: BAP (Brahma-associated proteins) and PBAP (Polybromo-associated BAP) [18] . In eukaryotes, translationally controlled tumour protein (TCTP) is a conserved protein involved in cancer and various cell functions in both cytoplasm and nucleus [19] , [20] , [21] , [22] , [23] , [24] , [25] . TCTP interacts with many cytoplasmic binding partners to participate in cell growth, proliferation, tumour invasion and apoptosis [19] , [20] , [26] , [27] . In addition, there is evidence that TCTP functions as a transcription factor [21] , [24] and a nuclear binding partner for ATM kinase during DNA repair [22] , [25] . In our previous study on the interaction between Drosophila TCTP (Tctp) and ATM for DNA repair, we observed that Tctp is widely distributed in interband regions of polytene chromosomes in salivary glands (SG). This prompted us to search for broader nuclear functions of Tctp at the level of chromatin. Here we show that Tctp binding to Brm antagonizes the Brm complex function to regulate gene transcription, transposon activation, and the stability of repeated sequences (rDNA and pericentromeric heterochromatin). Loss of Tctp causes a reduction of su(var)3-9 transcription, resulting in reduced H3K9me2/3 methylation. Our data suggest that Tctp regulates pericentromeric heterochromatin stability through histone modification and chromatin remodelling. This study provides new insights into the function of TCTP in genome stability and cancer. Tctp directly interacts and colocalizes with Brm Tctp is detected in the cytoplasm as well as in the nucleus ( Supplementary Fig. 1a ) where it is broadly distributed in the interband regions of polytene chromosomes from SG cells [22] . Since the interband regions are transcriptionally active with less-condensed euchromatic conformation [1] , it is possible that Tctp may play a role in the regulation of chromatin structure and transcription. Thus, we used yeast two-hybrid screen to identify novel Tctp-interacting partners and found a Brm polypeptide binding to Tctp ( Supplementary Fig. 1b ; Fig. 1a,c ). Brm is the catalytic ATPase subunit of the Brm chromatin remodeler involved in regulation of pericentromeric heterochromatin boundaries by antagonizing spreading of silencing and in transcriptional gene regulation [10] , [11] , [17] . The physical interaction between Tctp and Brm was reciprocally confirmed by co-immunoprecipitation (co-IP) using nuclear extracts from S2 cells transfected with FLAG-tagged full-length wild-type Brm (Brm WT ) and MYC-tagged Tctp ( Fig. 1b ). 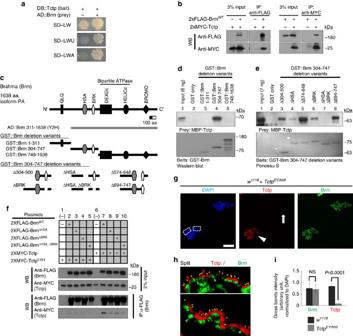Figure 1: Tctp physically interacts and colocalizes with Brm. (a) Y2H (yeast two-hybrid) assay. A functional Gal4 formed by direct interaction between Tctp bait and Brm prey activates the expression of Gal4-responsive selection markers (URA3andADE2), allowing yeast transformants to grow on the selection media SD-LWU (-uracil) or SD-LWA (–adenine). (b) Reciprocal co-IP. Brm (2xFLAG-BrmWT) is co-immunoprecipitated with Tctp (2xMYC-Tctp) in S2 cell andvice versa. (c–e)in vitroGST-Pull down assays. (c) Schematic domain structure of Brm and a list of mutated Brm polypeptide fragments used in pull-down assays. The full-length Brm protein has 6 conserved domains. (d) Direct Tctp binding to the middle part of Brm protein (304-747 amino-acid (aa) region, lane 4). (e) Both HSA and BRK domains of Brm are required for direct binding to Tctp (lane 4, 6, 7). (f) co-IP in S2 cell expressing 2xMYC-Tctp and 2xFLAG-full-length Brm with deletion of either HSA or BRK, or both domains. Deletion of either HSA or BRK domain of Brm reduces its interaction with Tctp (lanes 8, 9). Contrary toin vitropull down assay, BrmΔHSA,ΔBRKshows a weak interaction with Tctp (lane 10). TctpE12V(E12V substitution) substantially interferes with the binding between Tctp and Brm (Lanes 2-5). (g–j) Tctp colocalizes with Brm in SG polytene chromosomes. (g) Squashed polytene chromosomes from the mixed SG tissues of wild-type andTctpmutant larvae, stained with DAPI (blue), Tctp (red), and Brm antibodies (green). Scale bar, 50 μm. Contrary to wild-type chromosomes (red, arrowhead),TctpEY/h59mutant chromosomes show reduced staining with anti-Tctp antibody (arrow). (h) Enlarged split images of the two boxed regions of wild-type chromosomes shown ing. Most Tctp signals are colocalized with Brm (yellow arrowheads), but some areas show preferentially either Tctp (red arrowheads) or Brm (green arrowheads). (i) The quantified gross bands intensities of Tctp and Brm staining normalized to DAPI (n=10 SGs, mean±s.d.). NS, not significant (P=0.8). Figure 1: Tctp physically interacts and colocalizes with Brm. ( a ) Y2H (yeast two-hybrid) assay. A functional Gal4 formed by direct interaction between Tctp bait and Brm prey activates the expression of Gal4-responsive selection markers ( URA3 and ADE2 ), allowing yeast transformants to grow on the selection media SD-LWU (-uracil) or SD-LWA (–adenine). ( b ) Reciprocal co-IP. Brm (2xFLAG-Brm WT ) is co-immunoprecipitated with Tctp (2xMYC-Tctp) in S2 cell and vice versa . ( c – e ) in vitro GST-Pull down assays. ( c ) Schematic domain structure of Brm and a list of mutated Brm polypeptide fragments used in pull-down assays. The full-length Brm protein has 6 conserved domains. ( d ) Direct Tctp binding to the middle part of Brm protein (304-747 amino-acid (aa) region, lane 4). ( e ) Both HSA and BRK domains of Brm are required for direct binding to Tctp (lane 4, 6, 7). ( f ) co-IP in S2 cell expressing 2xMYC-Tctp and 2xFLAG-full-length Brm with deletion of either HSA or BRK, or both domains. Deletion of either HSA or BRK domain of Brm reduces its interaction with Tctp (lanes 8, 9). Contrary to in vitro pull down assay, Brm ΔHSA,ΔBRK shows a weak interaction with Tctp (lane 10). Tctp E12V (E12V substitution) substantially interferes with the binding between Tctp and Brm (Lanes 2-5). ( g – j ) Tctp colocalizes with Brm in SG polytene chromosomes. ( g ) Squashed polytene chromosomes from the mixed SG tissues of wild-type and Tctp mutant larvae, stained with DAPI (blue), Tctp (red), and Brm antibodies (green). Scale bar, 50 μm. Contrary to wild-type chromosomes (red, arrowhead), Tctp EY/h59 mutant chromosomes show reduced staining with anti-Tctp antibody (arrow). ( h ) Enlarged split images of the two boxed regions of wild-type chromosomes shown in g . Most Tctp signals are colocalized with Brm (yellow arrowheads), but some areas show preferentially either Tctp (red arrowheads) or Brm (green arrowheads). ( i ) The quantified gross bands intensities of Tctp and Brm staining normalized to DAPI ( n =10 SGs, mean±s.d.). NS, not significant ( P =0.8). Full size image In vitro pull-down assay using MBP-Tctp and GST-Brm deletion variants ( Fig. 1c ) revealed that Tctp directly binds to a 304–747 aa region of Brm ( Fig. 1d ) containing both HSA and BRK domains. Pull-down assays between MBP-Tctp and GST-Brm 304–747 deletion variants indicated that deletion of either HSA or BRK domain strongly reduced the binding between Brm and Tctp, while deletion of both domains abolished the binding of these two proteins. Thus, HSA and BRK domains are partially redundant, and loss of both domains critically impairs the binding between Brm and Tctp in vitro ( Fig. 1e , Lane 4, 6 and 7) compared with other parts of 304–747 aa region of Brm ( Fig. 1e , Lane 3, 5 and 8). Co-IP using S2 cells transfected with 2xMYC-Tctp and 2xFLAG-Brm variants also showed that deletion of either HSA or BRK domain significantly impaired the physical interaction between Tctp and Brm ( Fig. 1f , Lane 7–10). Interestingly, however, Brm deleted in both HSA/BRK domains still showed a weak binding to Tctp ( Fig. 1f , lane 10). Thus, although HSA and BRK domains are important for proper binding of these two proteins, a weak interaction may still be possible through another region of Brm in culture cells. Glutamate at the position 12 in the N-terminal region of Tctp is necessary for Tctp functions [22] , [26] . The interaction between Tctp and Brm was considerably reduced by the E12 substitution (E12 to V) (Tctp E12V ), indicating a role of E12 for binding between Tctp and Brm ( Fig. 1f , Lane 2–5). Consistent with these biochemical data, we also observed in vivo colocalization between Tctp and Brm in polytene chromosomes ( Fig. 1g,h ; Supplementary Fig. 2a ). To check the effects of Tctp mutation, chromosomes were prepared from a mixed SG samples of wild-type and Tctp EY /Tctp h59 trans-heterozygote (hereafter Tctp EY/h59 ). This trans-heterozygote provides a strong hypomorph condition [22] that can be identified by reduced Tctp expression. In Tctp-positive wild-type chromosomes, most Tctp colocalized with Brm within the interband regions ( Fig. 1g , arrowhead; Fig. 1h , yellow arrowheads), although some sites showed preferentially either Tctp or Brm ( Fig. 1h , red arrowheads for Tctp and green for Brm). In Tctp EY/h59 chromosomes, Tctp level was strongly reduced ( Fig. 1g , arrow), but Brm seemed to be intact at the gross level ( Fig. 1i ), although Tctp EY/h59 chromosomes showed minor variations in the Brm banding intensity ( Supplementary Fig. 2a , asterisks). Tctp knockdown by ptc-Gal4 ( ptc>Tctp-i ) also did not cause gross changes in the Brm level ( Supplementary Fig. 2c , white arrow). Similarly, Tctp levels were not changed significantly in polytene chromosomes with Brm silencing ( ptc>brm-i ) or dominant-negative Brm [28] expression ( ptc>Brm DN ) ( Supplementary Fig. 2d–e ). Additional tests with RNA interference (RNAi), mutant clones and overexpression conditions indicated that reduction or overexpression of Tctp does not alter the gross level of Brm and vice versa ( Supplementary Fig. 2f–l ). Taken together, our data indicate that Tctp and Brm directly bind to each other, and colocalize in most interband regions of chromosomes. Tctp negatively modulates Brm ATPase activity As shown above, Tctp loss does not greatly affect the level of Brm and vice versa in two different tissues. It led us to postulate that Tctp may interact with Brm to regulate the Brm activity rather than its recruitment. Previously, it has been shown that an HSA domain in yeast Sth1 or human Brg-1 ATPase subunit acts as the primary binding platform for nuclear actin-related proteins (ARPs) and β-actin (Act) and this interaction is required to facilitate maximum ATPase activity of the chromatin remodelers [29] , [30] . Since Tctp binds to the HSA domain of Brm and both Drosophila ARP4 and Act (ARP4/Act) also bind to the same domain ( Supplementary Fig. 3 ), we examined whether Tctp binding to the HSA domain might promote or interfere with ARP4/Act binding to Brm for regulating Brm ATPase activity. First, we performed co-IP in Tctp-knockdowned S2 cells coexpressing V5-ARP4, V5-act, and FLAG-Brm WT to observe the change in the binding affinity between Brm and ARP4/Act ( Fig. 2a ). Interestingly, ARP4/Act binding to Brm was increased by Tctp-knockdown ( Fig. 2a , arrows). This inverse relationship suggests that Tctp may negatively regulate Brm ATPase activity by interfering with ARP/Act binding to Brm. To attest this postulation, we assayed ATPase activity of Brm using immunoprecipitations in Tctp-knockdowned S2 cell nuclear extracts ( Fig. 2b–d ). Brm ATPase activity was measured at day 3 and 7 after dsRNA treatment. In vitro Brm ATPase activity was determined with a colorimetric Malachite green inorganic phosphate assay [31] , [32] , [33] . In this assay, immunoprecipitants from Tctp-knockdowned S2 cell extract ( Fig. 2c ) showed about 2.5-fold higher Brm ATPase activity than pSK(−) dsRNAi control ( Fig. 2d ). This result suggests that Tctp binding to Brm negatively modulates Brm ATPase activity by competing with ARP4/Act for binding to the HSA domain. 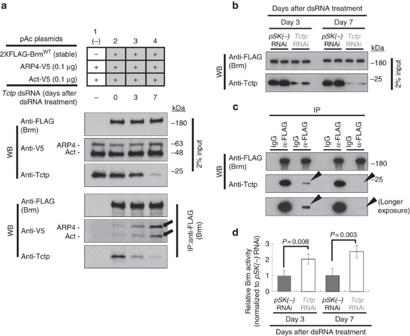Figure 2: Tctp binding to Brm negatively modulates Brm ATPase activity. (a) Enhanced ARP4/Act binding to Brm by Tctp reduction. V5-tagged ARP4 and Act were transiently expressed in S2 cells, stably transfected to produce 2XFLAG-BrmWT. Tctp-knockdown by RNA interference (RNAi) using double-stranded RNA (dsRNA) was treated twice at day 0 and 3 to maximize RNAi effect. Immunoprecipitation was performed using FLAG antibody. ARP4/Act binding to Brm was increased by Tctp reduction (arrows). (b–d)in vitroATPase activity assay in Tctp-knockdowned S2 cells. S2 cells were stably transfected to express 2xFLAG-BrmWT. (b) dsRNA was treated twice at day 0 and day3. (c–d) Brm immunoprecipitants from nuclear extracts with low levels of Tctp (arrowheads) were monitored for ATPase assay, relative to control precipitant (pSK(−)RNAi). (d) Brm ATPase activity was increased up to about 2.5-fold by Tctp-knockdown, compared withpSK(−)RNAi control. ATPase activity was normalized to that ofpSK(−)control.n=3 tests (mean±s.d.). Figure 2: Tctp binding to Brm negatively modulates Brm ATPase activity. ( a ) Enhanced ARP4/Act binding to Brm by Tctp reduction. V5-tagged ARP4 and Act were transiently expressed in S2 cells, stably transfected to produce 2XFLAG-Brm WT . Tctp-knockdown by RNA interference (RNAi) using double-stranded RNA (dsRNA) was treated twice at day 0 and 3 to maximize RNAi effect. Immunoprecipitation was performed using FLAG antibody. ARP4/Act binding to Brm was increased by Tctp reduction (arrows). ( b – d ) in vitro ATPase activity assay in Tctp-knockdowned S2 cells. S2 cells were stably transfected to express 2xFLAG-Brm WT . ( b ) dsRNA was treated twice at day 0 and day3. ( c – d ) Brm immunoprecipitants from nuclear extracts with low levels of Tctp (arrowheads) were monitored for ATPase assay, relative to control precipitant ( pSK(−) RNAi). ( d ) Brm ATPase activity was increased up to about 2.5-fold by Tctp-knockdown, compared with pSK(−) RNAi control. ATPase activity was normalized to that of pSK(−) control. n =3 tests (mean±s.d.). Full size image Tctp shows antagonistic genetic interaction with brm Biochemical data shown above indicate a negative relationship between Tctp and Brm. To determine whether Tctp and Brm are antagonistically related in vivo , we examined their genetic interactions in the wing. We took an advantage of the observation that Brm participates in wing vein formation by regulating EGFR signalling [34] , [35] . Brm overexpression by ap-Gal4 ( ap>brm ) in wing discs produced ectopic veins in both L2 and the posterior crossvein regions in about 60% of flies examined ( Fig. 3a ). This phenotype was considerably suppressed by co-expression of Tctp, but not by Tctp E12V ( Fig. 3a ). Interestingly, adult Tctp EY/h59 females also showed extra posterior crossvein phenotype (58% flies; Fig. 3b , black arrowheads), which was seen in only about 5% of adult females when brm 2 null heterozygote ( brm 2 /+) was introduced ( Fig. 3b , white arrowheads). This strong suppression implies that Brm activity increases in Tctp mutants, causing ectopic veins in the wing. These genetic interactions suggest that the physical interaction between Tctp and Brm ( Figs 1 and 2 ) is physiologically relevant. 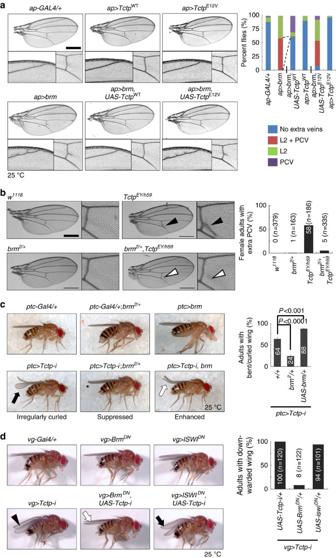Figure 3:Tctpis genetically antagonistic tobrm. (a) Genetic interaction of overexpressed Brm and Tctp. (Top)ap-Gal4/+,ap>Tctpandap>TctpE12Vdo not affect wing veins. Below each wing, regions of L2 vein and posterior crossvein (PCV) are shown at a higher magnification. (Bottom)ap>brmcauses ectopic veins near the L2 vein and the posterior crossvein. Co-expression of Tctp and Brm (ap>brm,Tctp) considerably suppresses the Brm overexpression phenotype. Overexpression of mutated TctpE12Vfails to suppress the Brm phenotype. (Histogram) Quantification of genetic interactions in percent flies. L2: extra veins in L2 vein. PCV: extra veins in the posterior crossvein. L2+PCV: extra veins in both.n=260-330 flies. Scale bar, 500 μm. (b) Genetic interaction betweenbrmandTctpmutations. Extra PCV (black arrowhead) phenotype in adultTctpEY/h59transheterozygotes is suppressed bybrm2/+ mutation (white arrowhead). (Histogram) Quantification of extra PCV phenotype in female adult flies. Scale bar, 500 μm. n=number of flies. (c) Antagonistic genetic interaction in wing shape. (Top)ptc-Gal4/+,ptc-Gal4/+;brm2/+ andptc>brmshow normal straight wings. (Bottom)ptc>Tctp-iflies show partial curled-up wings (black arrow). This phenotype is suppressed (asterisk) or enhanced (white arrow, curled-up wing) bybrmreduction or overexpression, respectively. (Histogram) Quantification of curled wing phenotype in adult flies (mean±s.d.).n=163–237 flies. (d) Genetic interaction betweenTctp-knockdown and dominant-negative Brm with catalytically inactive ATPase (BrmDN). (Top)vg-Gal4/+,vg>brmDN, andvg>ISWIDNshow normal straight wings. (Bottom) Downward-kinked adult wing phenotype ofvg>Tctp-iflies (black arrowhead) was suppressed by coexpressing BrmDN(white arrow), but not by ISWIDN(black arrow). ISWI is an ATPase subunit for other chromatin remodelers such as ACF, CHRAC, and NURF. (Histogram) Quantification of downward-kinked wing phenotype in adult flies. n=number of flies. Figure 3: Tctp is genetically antagonistic to brm. ( a ) Genetic interaction of overexpressed Brm and Tctp. (Top) ap-Gal4/+ , ap>Tctp and ap>Tctp E12V do not affect wing veins. Below each wing, regions of L2 vein and posterior crossvein (PCV) are shown at a higher magnification. (Bottom) ap>brm causes ectopic veins near the L2 vein and the posterior crossvein. Co-expression of Tctp and Brm ( ap>brm , Tctp ) considerably suppresses the Brm overexpression phenotype. Overexpression of mutated Tctp E12V fails to suppress the Brm phenotype. (Histogram) Quantification of genetic interactions in percent flies. L2: extra veins in L2 vein. PCV: extra veins in the posterior crossvein. L2+PCV: extra veins in both. n =260-330 flies. Scale bar, 500 μm. ( b ) Genetic interaction between brm and Tctp mutations. Extra PCV (black arrowhead) phenotype in adult Tctp EY/h59 transheterozygotes is suppressed by brm 2 /+ mutation (white arrowhead). (Histogram) Quantification of extra PCV phenotype in female adult flies. Scale bar, 500 μm. n=number of flies. ( c ) Antagonistic genetic interaction in wing shape. (Top) ptc-Gal4 /+, ptc-Gal4 /+; brm 2 /+ and ptc > brm show normal straight wings. (Bottom) ptc>Tctp-i flies show partial curled-up wings (black arrow). This phenotype is suppressed (asterisk) or enhanced (white arrow, curled-up wing) by brm reduction or overexpression, respectively. (Histogram) Quantification of curled wing phenotype in adult flies (mean±s.d.). n =163–237 flies. ( d ) Genetic interaction between Tctp -knockdown and dominant-negative Brm with catalytically inactive ATPase ( Brm DN ). (Top) vg-Gal4 /+, vg>brm DN , and vg>ISWI DN show normal straight wings. (Bottom) Downward-kinked adult wing phenotype of vg>Tctp-i flies (black arrowhead) was suppressed by coexpressing Brm DN (white arrow), but not by ISWI DN (black arrow). ISWI is an ATPase subunit for other chromatin remodelers such as ACF, CHRAC, and NURF. (Histogram) Quantification of downward-kinked wing phenotype in adult flies. n=number of flies. Full size image In addition, we confirmed the antagonistic relation between Tctp and brm using the phenotype of Tctp -RNAi induced by ptc-Gal4 . Adult wings of ptc>Tctp-i showed a weak curled-up phenotype (mildly curled or curling of only one wing; Fig. 3c , black arrow). The curled wing of ptc>Tctp-i was significantly suppressed or enhanced by Brm reduction or overexpression, respectively ( Fig. 3c , asterisk and white arrow), providing additional evidence for an enhanced Brm activity in the Tctp mutant background. The curled wing phenotype of ptc>Tctp-i flies was also modified by altered levels of positive modulators of Brm such as ARP4 (encoded by bap55 gene) and Act. Penetration of the weak curled-up wing phenotype in ptc>Tctp-i was considerably reduced to about 50% by heterozygous bap55 EY15967 or act cg0010 mutation. In contrast, overexpression of ARP4 or Act enhanced the curled-up wing phenotype marginally or considerably, respectively ( Supplementary Fig. 4a ). Hence, Tctp is antagonistically related to Brm and its associated regulators in development. To confirm the increased activation of the Brm function in Tctp mutants, we tested genetic interaction by coexpressing Tctp-i and Brm DN , a dominant-negative form deficient in ATPase activity due to K804R substitution in the ATP-binding site [28] . We used a vg-Gal4 driver to induce Brm DN expression in the dorsoventral boundary of wing disc ( Fig. 3d ). The downward-kinked adult wing phenotype of vg>Tctp-i flies was suppressed by coexpressing Brm DN , indicating that Tctp depletion causes activation of Brm function. This genetic interaction between Tctp silencing and Brm DN is specific because a dominant negative form of another class of chromatin remodeler ATPase, ISWI (ISWI DN , K159R substitution in the ATP-binding site) [36] showed no genetic interaction with vg>Tctp-i flies. Remarkably, high lethality in ptc>brm DN during mid-and late pupal stages ( Supplementary Fig. 4b , black arrows) was considerably suppressed or enhanced by Tctp-knockdown or overexpression, respectively ( Supplementary Fig. 4b , blue and red arrows). Collectively, these results indicate that Tctp is antagonistic to brm function in vivo , in accordance with the biochemical evidence for an inhibitory modulation of Brm ATPase activity by Tctp ( Fig. 2 ). Aberrant regulation of transcription in Tctp mutants In eukaryotes, Brm remodeler complexes are involved in transcriptional regulation of various target genes during development [11] , [14] , [16] , [18] , [35] , [37] , [38] , [39] , [40] . Especially, in Drosophila , PBAP complex physically interacts with the transcription initiation factor IID complex to make a single supercomplex in the promoter region for transcription start process [15] , [41] . In addition, Brm complex with a mutant form of inhibitory SNR1 subunit increases RNA polymerase II (Pol-II) elongation activity in Eig71E gene locus [37] , [40] . Direct interaction and antagonistic relation between Tctp and Brm led us to ask whether Tctp functions together with Brm to regulate transcription processes by changing the chromatin structure. First, we found that Tctp colocalizes with Pol-II in interband regions of polytene chromosomes ( Fig. 4a ). Interestingly, different Pol-II antibody markers (specific for the phosphorylation patterns of Pol-II C-terminal domain (CTD) during transcription) showed that most Tctp was colocalized with Pol-IIa of the pre-initiation complex at the promoter regions ( Fig. 4b ). Tctp was also localized with Pol-II Ser5 in the early transcription stage of promoter clearance ( Fig. 4c ) and Pol-II Ser2 in the late transcription stage ( Fig. 4d ). Consistent with these data, Pol-II antibody detecting both phosphorylated and non-phosphorylated CTD immunoprecipitated Pol-II with Brm and Tctp in S2 cell nuclear extract transfected with 2xFLAG-Brm WT and 2xMYC-Tctp ( Fig. 4e , left panels). Reciprocally, 2xMYC-Tctp or 2xFLAG-Brm was also immunoprecipitated with Pol-II, although the binding affinity was weak (longer exposures in Fig. 4e ). These data suggest that Tctp and the Brm complex may form a large protein complex with a transcription machinery to regulate the early transcription process. 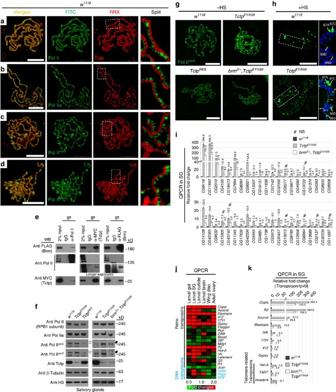Figure 4: Enhanced expression of a large set of genes and transposons inTctpmutants. (a–d) Tctp colocalizes with Pol-II in the interbands of squashed SG chromosome stained for Tctp and different CTD forms of the largest Pol-II subunit. (a) Staining with anti-Pol-II for non-phospho and phosphorylated CTD in all transcription steps. (b) anti-Pol-IIa for non-phosphorylated CTD in the promoter-recruited step. (c) anti-Pol-IISer5for Ser-5-phosphorylated CTD in transcription initiation. (d) anti-Pol-IISer2for Ser-2-phosphorylated CTD in transcription elongation. Boxed areas are enlarged as split images. Scale bars, 50 μm. (e) Co-IP using nuclear S2 cell extract transfected with both 2xFLAG-Brm and 2xMYC-Tctp. Tctp forms a large protein complex with Brm and Pol-II. These interactions are resistant to benzonase treatment suggesting direct interaction. The interaction between Tctp and Pol-II or Brm and Pol-II is relatively weak (longer exposures). (f) Effects of Tctp on transcription initiation and elongation in SG. Increased Pol-IISer5and Pol-IISer2levels inTctpEY/h59mutants (white arrows), which are restored by genomicTctpGe30-2in mutants (TctpRES) or by heterozygousbrm2mutation (black arrows). Note that the amount of Tctp inbrm2/+,TctpEY/h59is not restored. β-tubulin and Histone 3 (H3) are loading controls. (g,h) Chromosome localization of elongating Pol-II. (g) Pol-IISer2localization before heat-shock (-HS). (Top) Increased transcription elongation levels inTctpEY/h59, compared withw1118control. (Bottom) GenomicTctpGe30-2orbrm2/+rescues the high level of Pol-IISer2inTctpEY/h59. (h) Elongating Pol-II localization after heat-shock (+HS). (Top) Pol-IISer2in wild-type exclusively localizes to heat-chock loci after HS. Boxed heat-shock loci between 87 A and 95D are enlarged in the right. (Bottom) Substantial levels of Pol-IISer2inTctpmutants still remain at many euchromatic sites (white arrowheads). Scale bars, 50 μm. (i) QPCR. 34 of 42 genes with high expression levels inTctpmutants were suppressed bybrm2/+ mutation. (j,k) QPCR of transposon expression inTctpmutants. (j) Retrotransposons likeCopia,Blastopia,Gypsy, andR2are highly expressed in various tissues fromTctpEY/h59. (k) Additionalbrmmutation inTctpEY/h59(brm2/+,TctpEY/h59) suppresses the high level expression of transposons in SG (mean±s.d.).Het-A,TART, andInvader4are located in the telomere region. Figure 4: Enhanced expression of a large set of genes and transposons in Tctp mutants. ( a – d ) Tctp colocalizes with Pol-II in the interbands of squashed SG chromosome stained for Tctp and different CTD forms of the largest Pol-II subunit. ( a ) Staining with anti-Pol-II for non-phospho and phosphorylated CTD in all transcription steps. ( b ) anti-Pol-IIa for non-phosphorylated CTD in the promoter-recruited step. ( c ) anti-Pol-II Ser5 for Ser-5-phosphorylated CTD in transcription initiation. ( d ) anti-Pol-II Ser2 for Ser-2-phosphorylated CTD in transcription elongation. Boxed areas are enlarged as split images. Scale bars, 50 μm. ( e ) Co-IP using nuclear S2 cell extract transfected with both 2xFLAG-Brm and 2xMYC-Tctp. Tctp forms a large protein complex with Brm and Pol-II. These interactions are resistant to benzonase treatment suggesting direct interaction. The interaction between Tctp and Pol-II or Brm and Pol-II is relatively weak (longer exposures). ( f ) Effects of Tctp on transcription initiation and elongation in SG. Increased Pol-II Ser5 and Pol-II Ser2 levels in Tctp EY/h59 mutants (white arrows), which are restored by genomic Tctp Ge30-2 in mutants ( Tctp RES ) or by heterozygous brm 2 mutation (black arrows). Note that the amount of Tctp in brm 2/+ , Tctp EY/h59 is not restored. β-tubulin and Histone 3 (H3) are loading controls. ( g , h ) Chromosome localization of elongating Pol-II. ( g ) Pol-II Ser2 localization before heat-shock (-HS). (Top) Increased transcription elongation levels in Tctp EY/h59 , compared with w 1118 control. (Bottom) Genomic Tctp Ge30-2 or brm 2/+ rescues the high level of Pol-II Ser2 in Tctp EY/h59 . ( h ) Elongating Pol-II localization after heat-shock (+HS). (Top) Pol-II Ser2 in wild-type exclusively localizes to heat-chock loci after HS. Boxed heat-shock loci between 87 A and 95D are enlarged in the right. (Bottom) Substantial levels of Pol-II Ser2 in Tctp mutants still remain at many euchromatic sites (white arrowheads). Scale bars, 50 μm. ( i ) QPCR. 34 of 42 genes with high expression levels in Tctp mutants were suppressed by brm 2 /+ mutation. ( j , k ) QPCR of transposon expression in Tctp mutants. ( j ) Retrotransposons like Copia , Blastopia , Gypsy , and R2 are highly expressed in various tissues from Tctp EY/h59 . ( k ) Additional brm mutation in Tctp EY/h59 ( brm 2/+ , Tctp EY/h59 ) suppresses the high level expression of transposons in SG (mean±s.d.). Het-A , TART , and Invader4 are located in the telomere region. Full size image Next, we examined phosphorylation patterns of Pol-II CTD in SG from Tctp EY/h59 to check the effects of Tctp on Pol-II activity during transcription. Pol-II stability and Pol-II binding to promoter regions in Tctp EY/h59 seemed to be intact because the total amounts of Pol-II (RPB1 subunit) and promoter-recruited Pol-II (Pol-IIa) were similar to wild-type control ( Fig. 4f ), respectively. On the contrary, Pol-II activities in transcription initiation (Pol-II Ser5 ) and elongation (Pol-II Ser2 ) steps were considerably increased in Tctp EY/h59 , and the increased Pol-II activities were restored by introducing a wild-type Tctp genomic fragment ( Tctp G30e-2 ) ( Fig. 4f , white arrows). Notably, brm 2/+ mutation markedly suppressed the increased Pol-II activities in Tctp EY/h59 ( Fig. 4f , black arrows). These data suggest that Tctp is required to suppress a step of early transcription by negatively modulating Brm functions. These results were further confirmed by immunostaining of polytene chromosomes in Tctp EY/h59 . Pol-II activity in the transcription elongation step was higher in Tctp EY/h59 chromosomes than wild-type control ( Fig. 4g , top; Supplementary Fig. 5a–b ), while this phenotype was rescued by Tctp G30e-2 or a reduction of the Brm function (+/ brm 2 ) ( Fig. 4g , bottom; Supplementary Fig. 5c–d ). Heat-shock in larval stages is known to cause dynamic changes in Pol-II activity such as decreased elongating Pol-II in euchromatin interbands and then increase at several heat-shock loci [16] , [42] . Thus, we tested whether the Pol-II activity difference between wild-type and Tctp EY/h59 is still prominent after heat-shock treatment ( Fig. 4h ; Supplementary Fig. 5e–f ). After heat shock, active transcriptional elongation was exclusively restricted to heat-shock loci such as 87A, 93D and 95D in wild-type chromosomes ( Fig. 4h , top). Tctp EY/h59 also showed similar dynamic Pol-II activity changes, but a substantial fraction of Pol-II Ser2 was retained at a subset of euchromatic sites ( Fig. 4h , white arrowheads). Altogether, these results suggest that Tctp acts in a supercomplex containing the Brm complex and a transcriptional complex, and that in this large complex, Tctp may affect early transcription step and subsequent elongation process by negative modulation of Brm ATPase. Abnormally enhanced Brm and Pol-II activity in Tctp mutants suggested that Tctp may be required for proper gene transcription. This possibility was tested using mRNA expression profiles in SG cells from wild-type ( w 1118 ), Tctp h59/+ and Tctp EY/h59 ( Supplementary Fig. 6a–c ). A total of 1,765 genes with more than 1.5-fold differences compared with wild-type were used for heat-map analysis. As expected, expression of these genes was increased or decreased in proportion to the functional Tctp gene dosage ( Supplementary Fig. 6a ). In Tctp EY/h59 , about 55% of these genes (964/1,765) displayed increased expression levels, while 34% showed decreased levels (601/1,765) compared with the wild-type level. Gene Ontology analysis revealed that diverse functions of 1,315 genes are misregulated in Tctp EY/h59 with over 1.5-fold changes ( P <0.05) in their gene expression ( Supplementary Fig. 6b ; Supplementary Table 1 ). These gene functions were ranged from apoptosis, DNA repair, or neurogenesis to reproduction, although mRNA profiling was performed using SG tissue. Notably, quantitative PCR analysis (QPCR) on a subset of genes (42) with abnormal expression levels in Tctp EY /h59 revealed that the transcriptional levels of most of these genes (34/42) were considerably recovered by brm 2 /+ mutation ( Fig. 4i ), suggesting that abnormal transcription in Tctp mutants are likely due to an increase in the Brm function. Interestingly, we found that of 78 transposons arrayed in a DNA chip, 17 showed markedly elevated levels over 1.5-fold in Tctp EY/h59 , while 11 were reduced ( Supplementary Fig. 6c ). Uncontrolled transposon expression is known to cause various genome instability [43] , [44] , [45] , [46] . Notably, retrotransposons like R2 , Copia , and Accord located in pericentromeric regions [43] , [47] were highly expressed over 100-fold higher than wild-type. In addition, elevated expression of telomere-related TEs ( Invader4 and TART ) might be related to the telomere fusion phenotype found in Tctp mutants [22] . These abnormal transposon expressions were not tissue-specific because QPCR in various tissues from Tctp EY/h59 larvae (gut, SG, brain and wing disc) and adults (ovary) ( Fig. 4j and Supplementary Fig. 6d ) showed similar results, though transposon expression levels were relatively higher in endocycling tissues (gut, cuticle and SG) than mitotic tissues (brain, wing discs and ovary). These ectopic expressions of retrotransposons in Tctp EY/h59 were considerably reduced in brm 2 /+ , Tctp EY /h59 double mutants to about a half level of Tctp EY/h59 or the level comparable to wild-type control ( Fig. 4k ). These results suggest that Tctp may be required for proper silencing of genes and transposons by negatively modulating Brm activity. Defective position-effect variegation in Tctp mutants Retrotransposons are transcriptionally silenced by heterochromatic marks and associated proteins [2] , [3] , [46] . Because highly expressed transposons in Tctp EY /h59 are located in the pericentromeric region, ectopic expression of transposons in Tctp mutants may derive from loss of heterochromatin silencing. To test this assumption, we checked whether Tctp can affect position-effect variegation (PEV). PEV is a phenotypic variegation caused by random suppression of an euchromatic gene due to its abnormal juxtaposition to heterochromatin [48] . We utilized the PEV phenotype of In(1)w m4 ( Fig. 5a ), in which the white ( w ) gene is transposed close to pericentromeric heterochromatin on the X chromosome by a large inversion ( Supplementary Fig. 7a ) [49] , [50] . Due to PEV, w + expression is suppressed in w m4 /Y males, resulting in the formation of unpigmented or weakly pigmented regions in the eye ( Fig. 5a , black arrowhead). In control tests, the w m4 PEV phenotype was suppressed by a mutation in the su(var)2-5 gene encoding HP1a protein, one of the key proteins maintaining the heterochromatin structure. In contrast, this PEV phenotype was enhanced by a mutation in lid encoding a histone demethylase ( Fig. 5a ). We then examined the effects of Tctp mutations on PEV. Tctp heterozygous null mutation (+/ Tctp h59 ) considerably suppressed the w m4 phenotype, resulting in about 6-fold higher eye pigmentation than w m4 control eye ( Fig. 5a , white arrowhead). We also confirmed that Tctp h59/+ mutation increased the level of white gene transcription by about 2.5-fold in the w m4 line ( Supplementary Fig. 7b ). These data suggest that silencing of w m4 is compromised by Tctp mutation. 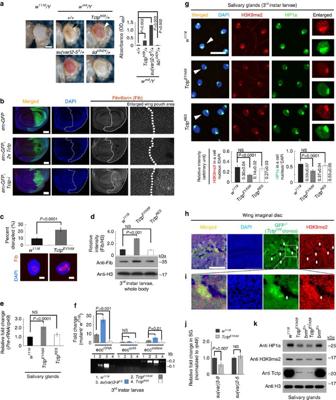Figure 5: Pericentromeric heterochromatin instability inTctpmutants. (a) Suppression ofwm4PEV phenotype byTctph59/+(white arrowhead). (Histogram) Quantification of eye pigment (n=20 heads, mean±s.d.). Scale bar, 200 μm. (b–f) Defective gene silencing and pericentromeric heterochromatin instability inTctpEY/h59mutants. (b) Effects of Tctp on expression ofrDNAgenes. Anen-Gal4was used to expressUAS-transgenes only in the posterior compartment of wing disc (dotted GFP-positive region). Fibrillarin (Fib) antibody staining for nucleolus is pseudo-colored in gray. (Top)en>GFPdiscs show similar Fib levels in both anterior and posterior compartments. (Middle) The reduced Fib level and nucleolar size in Tctp-overexpressing cells of the posterior compartment. (Bottom) The increased Fib level and nucleolar size in Tctp-knockdown cells of the posterior compartment. Scale bars, 50 μm. (c) Disrupted nucleolar structures in SG cells fromTctpEY/h59.n=30 SGs (mean±s.d.). Scale bars, 10 μm. (d) Elevated Fib levels inTctpEY/h59larvae.TctpRES(TctpEY/h59withTctpGe30-2) shows normal level of Fib. Anti-H3, a loading control for western blotting (mean±s.d.). NS (P=0.5). (e) IncreasedPre-rRNAtranscript from nucleolarrDNAloci inTctpEY/h59(QPCR).TctpRESrescuedTctpEY/h59(mean±s.d.). n.s. (P=0.5). (f) Increased eccDNA formation in the repeated genomic sequences such asrDNAandstellategenes ofTctpEY/h59.su(var)3-91/2, a positive control. QPCR was shown as a fold change relative to wild-type (mean±s.d.). A representative gel image is shown. NS (P=0.1). (g–k) Reduced level of H3K9me2 or HP1a heterochromatic silencing mark inTctpmutants. (g) (Top) High levels of silencing marks in SG nucleus from wild-type (w1118). (Right-most) The enlarged image of a nucleus marked by an arrowhead. (Middle) Reduced levels of silencing mark inTctpEY/h59. (Bottom)TctpGe30-2rescuesTctpEY/h59from reduced levels of silencing marks. Scale bar, 50 μm. (Histograms) Quantified silencing mark levels (n=10–14 SGs, mean±s.d.). NS (P=0.1). (h,i) Reduced H3K9me2 levels inTctph59null mitotic clones (GFP-negative, arrows) within the developing wing disc. The boxed region is enlarged ini. Scale bar, 50 μm. (j) QPCR in SG tissues. Reducedsu(var)3-9transcription inTctpEY/h59(mean±s.d.). NS (P=0.3). (k) Western blot on SG tissues. The levels of both H3K9me2 and HP1a inTctpEY/h59are reduced compared with wild-type. Figure 5: Pericentromeric heterochromatin instability in Tctp mutants. ( a ) Suppression of w m4 PEV phenotype by Tctp h59/+ (white arrowhead). (Histogram) Quantification of eye pigment ( n =20 heads, mean±s.d.). Scale bar, 200 μm. ( b – f ) Defective gene silencing and pericentromeric heterochromatin instability in Tctp EY/h59 mutants. ( b ) Effects of Tctp on expression of rDNA genes. An en-Gal4 was used to express UAS -transgenes only in the posterior compartment of wing disc (dotted GFP-positive region). Fibrillarin (Fib) antibody staining for nucleolus is pseudo-colored in gray. (Top) en>GFP discs show similar Fib levels in both anterior and posterior compartments. (Middle) The reduced Fib level and nucleolar size in Tctp-overexpressing cells of the posterior compartment. (Bottom) The increased Fib level and nucleolar size in Tctp-knockdown cells of the posterior compartment. Scale bars, 50 μm. ( c ) Disrupted nucleolar structures in SG cells from Tctp EY/h59 . n =30 SGs (mean±s.d.). Scale bars, 10 μm. ( d ) Elevated Fib levels in Tctp EY/h59 larvae. Tctp RES ( Tctp EY/h59 with Tctp Ge30-2 ) shows normal level of Fib. Anti-H3, a loading control for western blotting (mean±s.d.). NS ( P =0.5). ( e ) Increased Pre-rRNA transcript from nucleolar rDNA loci in Tctp EY/h59 (QPCR). Tctp RES rescued Tctp EY/h59 (mean±s.d.). n.s. ( P =0.5). ( f ) Increased eccDNA formation in the repeated genomic sequences such as rDNA and stellate genes of Tctp EY/h59 . su(var)3-9 1/2 , a positive control. QPCR was shown as a fold change relative to wild-type (mean±s.d.). A representative gel image is shown. NS ( P =0.1). ( g – k ) Reduced level of H3K9me2 or HP1a heterochromatic silencing mark in Tctp mutants. ( g ) (Top) High levels of silencing marks in SG nucleus from wild-type ( w 1118 ). (Right-most) The enlarged image of a nucleus marked by an arrowhead. (Middle) Reduced levels of silencing mark in Tctp EY/h59 . (Bottom) Tctp Ge30-2 rescues Tctp EY/h59 from reduced levels of silencing marks. Scale bar, 50 μm. (Histograms) Quantified silencing mark levels ( n =10–14 SGs, mean±s.d.). NS ( P =0.1). ( h , i ) Reduced H3K9me2 levels in Tctp h59 null mitotic clones (GFP-negative, arrows) within the developing wing disc. The boxed region is enlarged in i . Scale bar, 50 μm. ( j ) QPCR in SG tissues. Reduced su(var)3-9 transcription in Tctp EY/h59 (mean±s.d.). NS ( P =0.3). ( k ) Western blot on SG tissues. The levels of both H3K9me2 and HP1a in Tctp EY/h59 are reduced compared with wild-type. Full size image Besides w m4 allele, Tctp mutation also suppressed PEV phenotypes of two additional lines, T(2;3)Stubble Variegated ( Sb v ) and Tp(3:Y)BL2 ( Supplementary Fig. 7c–d ). In Sb v , a defined chromatin region near the Sb gene is translocated by the centromeric heterochromatin region of the 2nd chromosome, which causes shortening of 1 or 2 scutellar macrochaete bristles by PEV. Tctp h59 /+ significantly increased the number of shortened scutellum bristles in Sb V line (about 1.8-fold compared with +/+ control; Supplementary Fig. 7c ). In Tp(3;Y)BL2/+ , a HS-lacZ transgene inserted in the euchromatic region of the third chromosome (65E) [48] , [49] is transposed to the heterochromatic Y chromosome [9] , leading to a strong suppression of LacZ expression by PEV in the SG. Both +/ Tctp h59 and +/ Tctp EY09182 increased the number of SG cells expressing LacZ in BL2 line ( Supplementary Fig. 7d , about 7-fold increase compared with +/+ control). Both cases of PEV suppression by Tctp mutants were fully restored by introducing Tctp Ge30 -2 ( Supplementary Fig. 7c–d ). Altogether, these results strongly suggested that Tctp is required to maintain pericentromeric heterochromatin silencing or boundaries. Instability of the repeated sequences in Tctp mutants In eukaryotic genome, silencing histone marks protects repetitive sequences (such as ribosomal RNA genes ( rDNA )) and pericentromeric repeats by inhibiting recombination between DNAs with similar sequences. In addition, transcriptional silencing of specific genes such as rDNA and transposons prevents cell lethality caused by excessive gene/transposon expression [8] , [51] . Since tandemly-repeated rRNA genes are proximal to pericentromeric heterochromatin region and their expression is partially suppressed by silencing histone marks [9] , we addressed whether rRNA gene silencing and rDNA structure are impaired in Tctp mutants. First, we checked Fibrillarin protein level (Fib; an RNA-binding protein for efficient processing of Pre‐rRNA in nucleolus) in Tctp-knockdowned wing discs from en>Tctp-i larvae. These discs showed considerably increased Fib protein levels and nucleolar size in the posterior region ( Fig. 5b , bottom) compared with the anterior compartment of the same disc or en>GFP control. Tctp overexpression in the posterior compartment showed a marginal reduction in the Fib level ( Fig. 5b , middle). In SGs, the nucleolar morphology was also disrupted with about 2-fold increase in the Fib-positive areas in Tctp EY/h59 ( Fig. 5c ), suggesting abnormal repair of double-strand breaks (DSBs) in these sequences [6] . Furthermore, the Fib protein level in the whole body from Tctp EY/h59 was increased about 2.9-fold ( Fig. 5d ). Consistent with these results, QPCR of rRNA transcription in SG showed about 2-fold increase in Tctp EY/h59 ( Fig. 5e ). During normal development, tandemly repeated sequences often make extrachromosomal circular DNA (eccDNA) through intramolecular homologous recombination between tandem repeats, causing genome instability. This eccDNA formation is markedly increased when genome is exposed to mutagens causing DSBs or when heterochromatin formation is defective by su(var)3-9 1/2 mutation ( Fig. 5f ) [6] , [51] . Interestingly, Tctp EY/h59 showed an increased eccDNA formation from the tandem-repeats such as rDNA (9.5-fold) and stellate (encoding casein kinase beta subunit; 2.9-fold) genes ( Fig. 5f ). The stellate locus is located in the pericentromeric heterochromatin of chromosome X [9] . Reduced gene silencing and increased eccDNA in Tctp EY/h59 were restored to the wild-type level by introducing Tctp Ge30-2 ( Tctp RES in Fig. 5d–f ). These results suggest that Tctp is required to maintain the stability of rDNA loci and pericentromeric repeated sequences. Reduced heterochromatic silencing components in Tctp mutants H3K9me2/3 histone modification catalysed by SU(VAR)3-9 HMT is an essential step for the recruitment of HP1a, leading to heterochromatin formation or gene silencing in Drosophila . Thus, H3K9 methylation and HP1a are convenient markers for silencing associated with heterochromatin structure [3] , [6] , [8] , [46] . Since mutations in Tctp and su(var)3-9 result in similar induction of eccDNAs in rDNA and heterochromatic sequences [6] , we assessed whether su(var)3-9 and other silencing components are affected in Tctp mutants. Indeed, larval SG tissues from Tctp EY/h59 or Sgs3>Tctp-i showed considerably reduced levels of H3K9me2 and HP1a ( Fig. 5g ; Supplementary Fig. 7g ). In cell nucleus from Tctp EY/h59 , H3K9me2 level was reduced to about 47% of wild-type ( Fig. 5g ). Likewise, polytene chromosomes from SGs of Tctp EY/h59 showed about 63% reduced H3K9me2 levels in the chromocenter ( Supplementary Fig. 7e–f ). Consistent with these results, both the mitotic Tctp h59 null clonal cells of wing disc and the posterior compartment of en>Tctp-i wing discs showed strong reduction in the levels of H3K9me2 ( Fig. 5h,i ) and H3K9me3 ( Supplementary Fig. 7i , arrowhead), respectively. In addition, HP1a levels were reduced in cell nuclei and polytene chromosomes from Tctp EY/h59 ( Fig. 5g ; Supplementary Fig. 7e–f ). The reduction of silencing marks in Tctp mutants was restored by introducing Tctp Ge30-2 ( Fig. 5g and Supplementary Fig. 7e , Tctp RES ). The reduction of silencing marks in Tctp mutants appears to result from the decreased amounts of SU(VAR)3-9 HMT protein, rather than the decreased enzyme activity for three reasons. Firstly, su(var)3-9 transcription was reduced in Tctp EY/h59 to about a half of the wild-type level ( Fig. 5j ). Secondly, chromatin IP assays revealed that Pol-II accumulation to su(var)3-9 locus was reduced in Tctp-knockdowned S2 cells to about 47% of pSK(-) RNAi control ( Supplementary Fig. 8d ). Finally, direct interaction among Tctp, SU(VAR)3-9, and HP1a was not detected in our assay (data not shown). Notably, transcription of su(var)2-5 gene encoding HP1a in Tctp EY/h59 was intact, although its protein level was decreased ( Fig. 5j,k ). This suggests that the stability of HP1a protein might be reduced in Tctp mutants by the decreased level of SU(VAR)3-9 protein. We also checked whether the effects of Tctp mutations on the level of silencing marks are related to an increase in the Brm function. Interestingly, the reduced levels of H3K9me2 and HP1a in Tctp EY/h59 were not restored by brm 2 /+ ( Fig. 5k ). Furthermore, the level of Brm in the su(var)3-9 locus was very low and unchanged by Tctp-knockdown ( Supplementary Fig. 8f ). Overall, these results suggest that Tctp is required for su(var)3-9 transcription, thus affecting the levels of H3K9 methylation and HP1a. These are likely to contribute to the formation of eccDNA in rDNA and pericentromeric heterochromatin. In this process, Tctp mutants are not affected at least by partial reduction of Brm. Brm reduction suppresses genome instability in Tctp mutant Heterozygote for brm 2 mutation can enhance PEV or TPE (telomeric position effect) phenotype by increasing heterochromatin-mediated suppression of w + expression in adult male [17] , [52] , [53] . Because Tctp and Brm directly interact each other and are biochemically and genetically antagonistic, we addressed whether the suppression of w m4 PEV phenotype in Tctp h59/+ may be restored by brm 2 mutation. Indeed, we found that brm mutation (+/ brm 2 ) strongly suppressed the effects of Tctp mutation ( Tctp h59 /+) on the w m4 PEV phenotype ( Fig. 6a , black arrow and histogram). Consistent with this, core subunit genes of the Brm complex such as mor and snr1 also interacted genetically with Tctp in the w m4 background. Heterozygous mor mutation (+/ mor 1 ), a known w m4 -enhancer, reduced eye pigmentation of Tctp h59/+ ( Fig. 6a , white arrowhead), while a known w m4 -suppressor, heterozygous snr1 mutation (+/ snr1 101319 ), increased eye color ( Fig. 6a , black arrowhead). These data suggest that pericentromeric heterochromatin instability in Tctp mutants is related to an abnormal activation of the Brm complex function, although the reduced levels of the silencing marks, H3k9me2/3 and HP1a in Tctp EY/h59 were not restored by brm 2 /+ mutation. 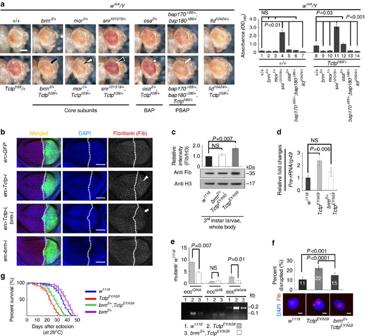Figure 6: Defective gene silencing and genome stability inTctpmutants are ameliorated bybrmmutation. (a) Genetic interaction between Tctp and Brm complex subunit genes. (Top panels)wm4eye color PEV phenotype in the wild-type background (+/+) and the effects of mutations in Brm complex genes as indicated.lid10424is a PEV enhancer control. (Bottom panels)Tctph59/+ heterozygous mutation strongly suppresses thewm4PEV (asterisk in the first panel). The effects ofTctph59/+ is significantly suppressed bybrm2/+mutation (black arrow). Likewise,mor1/+ (white arrowhead) andbap170Δ65/+;bap180Δ86/+ double mutations (PBAP components, white arrow) suppress theTctph59/+ effect. In contrast,snr101319/+ mutation in an inhibitory subunit gene (black arrowhead) orosa2/+ (BAP component) does not suppressTctph59/+. Scale bar, 200 μm. (Histogram) Quantification of eye pigment (Mean±s.d.n=20 heads). (b,c) Increased Fib levels inTctpmutants. (b) Increased Fib level in the posterior compartment ofen>Tctp-iflies (arrowhead) is suppressed by Brm-knockdown (arrow). Scale bars, 50 μm. (c) Increased Fib level inTctpEY/h59whole body. Fib (nucleolus marker) and H3 (loading control) antibodies were used for western blotting or immunostaining. (d,e) QPCR onPre-rRNAtranscription and eccDNA formation. Additional heterozygousbrm2mutation inTctpEY/h59ameliorates defective gene silencing inrDNAloci from SG cell nucleoli (d) and larval eccDNA formation in repetitive sequences (e). Normalized DNA levels are shown as fold changes relative to the wild-type level (mean±s.d.). A representative gel image is shown. (f) Abnormal nucleolar morphology inTctpEY/h59are improved bybrm2/+ mutation. Scale bars, 10μm. (g) Shortened life span in adultTctpEY/h59males (red) relative to wild-type (blue; log-rank test,P<0.0001) is ameliorated by reducing Brm level (brm2/+,TctpEY/h59; green; log-rank test,P<0.0001). Adult flies were incubated at 29 °C. Figure 6: Defective gene silencing and genome stability in Tctp mutants are ameliorated by brm mutation. ( a ) Genetic interaction between Tctp and Brm complex subunit genes. (Top panels) w m4 eye color PEV phenotype in the wild-type background (+/+) and the effects of mutations in Brm complex genes as indicated. lid 10424 is a PEV enhancer control. (Bottom panels) Tctp h59 /+ heterozygous mutation strongly suppresses the w m4 PEV (asterisk in the first panel). The effects of Tctp h59 /+ is significantly suppressed by brm 2/+ mutation (black arrow). Likewise, mor 1 /+ (white arrowhead) and bap170 Δ65 /+; bap180 Δ86 /+ double mutations (PBAP components, white arrow) suppress the Tctp h59 /+ effect. In contrast, snr 101319 /+ mutation in an inhibitory subunit gene (black arrowhead) or osa 2 /+ (BAP component) does not suppress Tctp h59 /+. Scale bar, 200 μm. (Histogram) Quantification of eye pigment (Mean±s.d. n =20 heads). ( b , c ) Increased Fib levels in Tctp mutants. ( b ) Increased Fib level in the posterior compartment of en>Tctp-i flies (arrowhead) is suppressed by Brm-knockdown (arrow). Scale bars, 50 μm. ( c ) Increased Fib level in Tctp EY/h59 whole body. Fib (nucleolus marker) and H3 (loading control) antibodies were used for western blotting or immunostaining. ( d , e ) QPCR on Pre-rRNA transcription and eccDNA formation. Additional heterozygous brm 2 mutation in Tctp EY /h59 ameliorates defective gene silencing in rDNA loci from SG cell nucleoli ( d ) and larval eccDNA formation in repetitive sequences ( e ). Normalized DNA levels are shown as fold changes relative to the wild-type level (mean±s.d.). A representative gel image is shown. ( f ) Abnormal nucleolar morphology in Tctp EY/h59 are improved by brm 2 /+ mutation. Scale bars, 10μm. ( g ) Shortened life span in adult Tctp EY/h59 males (red) relative to wild-type (blue; log-rank test, P <0.0001) is ameliorated by reducing Brm level ( brm 2/+ , Tctp EY/h59 ; green; log-rank test, P <0.0001). Adult flies were incubated at 29 °C. Full size image In most eukaryotes including flies, Brm-containing chromatin remodelers are divided into two subclasses according to their specific accessary subunits, BAP (SWI/SNF in yeast and BAF in mammals) and PBAP (RSC in yeast and PBAF in mammals; Fig. 7a ). BAP contains OSA, whereas PBAP has Bap170, 180 and SAYP. Tctp h59/+ showed strong genetic interaction with double heterozygous mutations of bap170/180 (+/ bap170 Δ65 ;+/ bap180 Δ86 ) in the w m4 background, resulting in suppression of the Tctp mutation effects ( Fig. 6a , white arrow). In contrast, the Tctp mutant effects were not modified by heterozygous osa mutation (+/ osa 2 ; Fig. 6a , square). Thus, Tctp seems to interact more preferentially with PBAP than BAP to facilitate pericentromeric heterochromatin silencing. 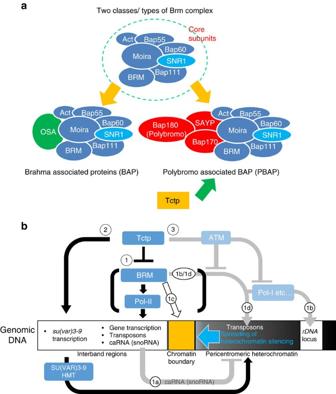Figure 7: Genetic interaction between Tctp and PBAP and a model for nuclear Tctp function for genome stability. (a) The schematic drawing of Brm chromatin remodelling complexes. Brm-containing chromatin remodelers can be divided into two types: BAP and PBAP according to their specific subunits, OSA and Bap160/170/SAYP, respectively. Based on genetic interactions (Fig. 6), Tctp seems to preferentially interact with PBAP than BAP. (b) A schematic model of novel nuclear Tctp functions for the stability of repeated sequences (rDNAand pericentromeric heterochromatin). Note thatrDNAlocus is not a part of heterochromatin although it is proximal to or surrounded by pericentromeric heterochromatin. Tctp keeps the stability of repeated sequences through three possible mechanisms: (Step 1) Tctp inhibits excess Brm activity, thereby regulating proper transcription level of various genes including transposons and stabilizing pericentromeric heterochromatin. caRNA expression and Pol-I activity regulated by Brm may also affect stability of pericentromeric heterochromatin (Step 1a and 1b, respectively). Brm may regulate the chromatin boundary (Step 1c). It might also be possible that Tctp mutations affect PEV by elevating the Brm activity within the regions of pericentromeric heterochromatin (Step 1d). (Step 2) Tctp positively regulatessu(var)3-9transcription by direct binding tosu(var)3-9locus, facilitating H3K9 methylation in pericentromeric regions. (Step 3) Brm or Pol-I may also be suppressed by the interaction between Tctp and ATM. See Discussion for details. Figure 7: Genetic interaction between Tctp and PBAP and a model for nuclear Tctp function for genome stability. ( a ) The schematic drawing of Brm chromatin remodelling complexes. Brm-containing chromatin remodelers can be divided into two types: BAP and PBAP according to their specific subunits, OSA and Bap160/170/SAYP, respectively. Based on genetic interactions ( Fig. 6 ), Tctp seems to preferentially interact with PBAP than BAP. ( b ) A schematic model of novel nuclear Tctp functions for the stability of repeated sequences ( rDNA and pericentromeric heterochromatin). Note that rDNA locus is not a part of heterochromatin although it is proximal to or surrounded by pericentromeric heterochromatin. Tctp keeps the stability of repeated sequences through three possible mechanisms: (Step 1) Tctp inhibits excess Brm activity, thereby regulating proper transcription level of various genes including transposons and stabilizing pericentromeric heterochromatin. caRNA expression and Pol-I activity regulated by Brm may also affect stability of pericentromeric heterochromatin (Step 1a and 1b, respectively). Brm may regulate the chromatin boundary (Step 1c). It might also be possible that Tctp mutations affect PEV by elevating the Brm activity within the regions of pericentromeric heterochromatin (Step 1d). (Step 2) Tctp positively regulates su(var)3-9 transcription by direct binding to su(var)3-9 locus, facilitating H3K9 methylation in pericentromeric regions. (Step 3) Brm or Pol-I may also be suppressed by the interaction between Tctp and ATM. See Discussion for details. Full size image Antagonistic interaction between Tctp and Brm in w m4 PEV phenotype suggested that abnormally enhanced function of Brm in Tctp mutants may exacerbate the stability of silenced repeated sequences. We tested this possibility in brm and Tctp double mutant or RNAi conditions ( Fig. 6b–f ). As expected, various characteristics of genome instability in Tctp mutants, including elevated rDNA expression, abnormal nucleolar morphology, and eccDNA formation, were ameliorated by reducing Brm activity in the double mutant condition (brm 2/+ , Tctp EY/h59 or en>Tctp-i,brm-i ). Increased Fib level in en>Tctp-i or Tctp EY/h59 was considerably suppressed by Brm-knockdown ( UAS-brm-i ) or brm 2 /+ mutation, respectively ( Fig. 6b,c ). Consistent with this, increased Pre-rRNA expression, eccDNA formation and disrupted nucleolar morphology in Tctp EY/h59 were also suppressed by brm 2 /+ mutation ( Fig. 6d–f ). It has been shown that increased transposon expression causes life span reduction by de novo insertional mutations or mRNA toxicity [45] . Similarly, adult Tctp EY/h59 males showed a shortened life span (32.8±1.5-d-old) compared with wild-type (43.8±2.1 days) at 29 °C ( Fig. 6g ). This phenotype was improved by 5.4 days in the presence of brm 2/+ (38.2±1.7 days), suggesting that the reduced life span in Tctp EY/h59 might be due to increased Brm function to some extent. Heterochromatin silencing has important roles in the maintenance of genome stability. Silencing histone marks prevents transposon jumping and abnormal recombination between repetitive sequences ( rDNA and pericentromeric heterochromatin), thereby restraining structural lesions in chromosomal DNA. Here we have shown a multitude of evidence that Tctp is required to stabilize pericentromeric heterochromatin in concert with Brm remodeler and to regulate su(var)3-9 histone gene transcription for producing histone marks for silencing. Tctp physically interacts with Brm, providing the basis for their genetic interaction. Tctp and Brm proteins also show extensive co-localization in the interband regions of polytene chromosomes and they work antagonistically in the regulation of gene expression. Analysis of chromosomal localizations in Tctp or brm mutant SGs indicates that Tctp is not critically required for the localization of Brm and vice versa at the gross level. This suggests that the physical interaction between Tctp and Brm might be involved in the regulation of their activity rather than their chromosomal localization. In fact, Tctp knockdown results in strong upregulation of the ATPase activity of Brm, suggesting that an important function of Tctp is to inhibit the ATPase activity of Brm. Precise mechanism for the Tctp-mediated inhibition of the Brm ATPase activity is currently unknown. However, we have shown that reduced Tctp facilitates binding of both ARP4 and Act to the HSA domain of Brm. Hence, Tctp seems to antagonize the Brm ATPase activity by competitively interfering with the binding of ARP4 and Act. The biochemical evidence for the Tctp function of inhibiting the Brm activity is strongly supported by antagonistic genetic interactions between Tctp and brm in multiple organs like eye, wing and SG, and even in the survival rate of adult flies. Hence, Tctp and Brm antagonistically affect gene expression and developmental events as well as adult life of flies. In addition to its antagonistic role with Brm, Tctp is required for the expression of Su(var)3-9 HMT, thus promoting H3K9 methylation and pericentromeric heterochromatin silencing and stability. On the basis of these findings, we propose a model for the functions of Tctp in the regulation of transcription, heterochromatin silencing, and the stability of repeated sequences ( Fig. 7b ). In this simplified scheme, Tctp regulates gene transcription and heterochromatic stability. To stabilize repeated sequences, Tctp plays two related functions: a negative regulation of Brm activity and a positive regulation of su(var)3-9 expression, the step (1) and (2) in Fig. 7b , respectively. In the step 1, Drosophila Brm participates in the processes for gene transcription [14] , [16] , [35] , [37] , [39] and the inhibition of heterochromatin spreading [17] , [52] , [53] . Our data show that both of these Brm functions are negatively regulated by Tctp. For example, Tctp is necessary for suppressing excessive or unwanted transcription of heterochromatic genes like transposons and for preventing eccDNA formation or heterochromatin spreading by suppressing the Brm remodeler activity. The role of Tctp in regulating the transcription of repair genes such as Ku70/80 and tefu might in part account for the instability of repeated sequences observed in the absence of Tctp. Our data for the role of Tctp in stabilizing the pericentromeric heterochromatin may also be explained by the inhibitory function of Tctp to Brm (step 1, Fig. 7b ). Interestingly, transcription of some snoRNA molecules including chromatin-associated RNA (caRNA; CR34558, CR34684, and CR33674) is upregulated in Tctp mutants, and these effects are suppressed by brm mutation ( Supplementary Fig. 11 ). Hence, Tctp might be involved in inhibiting the Brm function of producing small ncRNAs (non-coding RNAs) such as snoRNA or caRNA. Small ncRNA including snoRNA and small interfering RNA have important roles in the formation of heterochromatin or gene silencing in eukaryotes [54] , [55] . Especially, since caRNA is a mediator for the establishment of open chromatin states in flies and humans [56] , increased Brm function might affect pericentromeric silencing via caRNA (step 1a, Fig. 7b ). It is also worth noting that in mammals, human Brm homologues can interact with nucleolar proteins [57] , [58] , [59] . Thus, uncontrolled Brm access to the nucleolus in Tctp mutant cells might affect rDNA instability via interacting with Pol-I or other components, as indicated by the step 1b in Fig. 7b . Brm chromatin remodeler can also affect pericentromeric heterochromatin by regulating the chromatin boundary in Drosophila [17] , [52] (step 1c, Fig. 7b ). In this process, Brm works together with the GAGA-FACT-HIRA complex for Histone3.3 (H3.3) replacement at the chromatin boundary, thereby inhibiting the spreading of hetrochromatin silencing [17] . However, it has been unknown how Brm function at the boundary is regulated. In this regard, it is noteworthy that Tctp mutants show abnormal PEV. This defect is considerably suppressed by reducing the brm gene dosage. Our data suggest that Tctp may negatively regulate Brm function at the chromatin boundary. However, since localization of PBAP subunits or ASF1 interacting with Brm is also detected in the regions of pericentromeric heterochromatin [60] , [61] , [62] , we do not exclude the possibility that Tctp mutations may affect PEV by elevating the Brm activity within the regions of pericentromeric heterochromatin (Step 1d). In addition to the function of Tctp through its interaction with Brm, we also propose an additional mechanism of Tctp in controlling the stability of pericentromeric heterochromatin. In this pathway (step 2, Fig. 7b ), Tctp is required for histone modification by regulating su(var)3-9 expression. Our data show that both levels of su(var)3-9 HMT transcription and H3K9me2/3 silencing mark are reduced in Tctp mutants. Further, ChIP analysis also supports that Tctp may function as a positive transcriptional modulator to mediate Pol-II accumulation on the su(var)3-9 locus. Because Tctp-dependent regulation of su(var)3-9 transcription is not modified by brm mutation, Tctp appears to regulate the expression of su(var)3-9 in a Brm-independent manner. Although Tctp can directly bind to su(var)3-9 locus for positive regulation, the precise role of Tctp for transcription control of su(var)3-9 is currently unknown. However, because mammalian TCTP regulates transcription of oct4 / nanog genes [21] , [24] , Drosophila Tctp might function as a transcription factor or a transcriptional regulator for su(var)3-9 . It is also possible that like Drosophila SNR1 (ref. 40 ), Tctp might regulate the stability of su(var)3-9 transcript during transcriptional elongation process. Our findings show that Tctp contributes to the stability of heterochromatin by its physical interaction with Brm. Previous studies have shown that Tctp directly interacts with ATM-kinase to promote DNA damage repair in Drosophila and mammalian cells [22] , [25] . Interestingly, ATM is also known to inhibit local Pol-II and pan-nuclear Pol-I activities in response to DSB [63] , [64] . Thus, it raises a question whether impaired ATM activity resulting from reduced Tctp might be responsible for increased Pol-II and Pol-I activity in Tctp mutants. Our tests for this possibility indicated that, in the absence of DSB induction, loss of ATM does not increase Pol-II activity in developing tissues of Drosophila and only leads to a weak increase in the Pol-I activity ( Supplementary Fig. 9a and Supplementary Discussion for details). It has been reported that mammalian Brm homologs like hBrm and Brg-1 act together with ATM to repair IR-induced DSBs at γ-H2AX foci [65] . Unlike Tctp, however, Drosophila Brm shows little co-localization with γ-H2Av foci, and reduced Brm does not affect the level of γ-H2Av, suggesting that ATM might not work together with Brm for DNA repair in developing organs of Drosophila ( Supplementary Fig. 10 and Supplementary Discussion ). On the other hand, we noted that heterozygous atm mutation can suppress w m4 PEV phenotype ( Supplementary Fig. 9b , arrow), and this suppression is significantly counteracted by brm heterozygous mutation ( Supplementary Fig. 9b , black arrowhead). Since this genetic interaction between atm and brm is similar to that of between Tctp and brm , it appears that Tctp-ATM complex might negatively regulate Brm function to stabilize heterochromatin boundaries or epigenetic modifications ( Fig. 7b , Step 3). However, genetic interaction between Tctp and ATM in w m4 + PEV might be additive rather than synergistic ( Supplementary Fig. 9b , white arrowhead). Thus, it is possible that Drosophila ATM and TCTP might function in parallel pathways to promote heterochromatin silencing or the establishment of its boundaries by negatively regulating Brm activity. Further studies are necessary to understand the precise relationship between ATM and TCTP. Nonetheless, our data suggest critical roles of Tctp in antagonizing the Brm function for the regulation of gene transcription and genome stability, providing insights into possible similar functions of human TCTP. Fly stocks and genetics All crosses were carried out at 25 °C on standard cornmeal media unless otherwise specified. w 1118 flies were used as the wild-type. Fly stocks of Sb V (BL878), In(1)w m4 ; su(var)2-5 5 (BL6234), su(var)3-9 1 (108-675), su(var)3-9 2 (108-676), lid 10424 (BL12367), Sgs3-Gal4 (BL6870; SG-specific Gal4 driver), ptc-Gal4 (BL2017), MS1096-Gal4 (BL8860), UAS-brm (BL42229), UAS-brm-RNAi ( brm-i , BL31712), mor 1 (107-129), snr 101319 (BL11529), osa 2 (107-130), bap55 EY15967 (BL21174) act5C cg0010 (BL12083), UAS-act5C (BL24779), Ay-Gal4 (107724) and brm 2 (107-133) were from the Bloomington Drosophila stock center (Bloomington, USA), DGRC (Kyoto, Japan), or VDRC (Vienna, Austria). w m4 was segregated from BL6234 and outcrossed to the w 1118 . Heterozygous su(var)2-5 5 and lid 10424 mutants are used as controls for PEV suppressor and enhancer, respectively. Fly stocks of P[w + ,HS-lacZ]65E and Tp(3;Y)BL2 (Joel C. Eissenberg, St Louis University), UAS-HA- tagged brm DN and UAS-ISWI DN (Fengwei Yu, National University of Singapore [23] ), bap170 Δ65 bap180 Δ86 and brm T362 (Jessica Treisman, New York University [14] ) were generous gifts. Tctp h59 , Tctp EY09182 , genomic rescue transgene Tctp Ge30-2 , UAS-Tctp-RNAi ( Tctp-i ), UAS-Tctp , and UAS-Tctp E12V were as reported previously [26] . Tctp EY/h59 strong hypomorphs were generated by crossing Tctp EY09182 /TM6b and Tctp h59 /TM6b flies [22] . ptc-Gal4 (second chromosome insertion) is used to express UAS -transgenes in SG tissue and AP boundary of wing discs. Mutant clones were induced using the FLP/FRT system [66] . Larvae were heat-shocked for 1 h at 38 °C at either 24 h ( Tctp EY09182 clone), 72 h ( brm T362 clone), or 96 h ( Tctp h59 clone) after egg deposit in the following genotypes: hs-FLP / (+ or Y ); FRT82B, Ubi-nGFP/FRT82B, Tctp EY09182 , hs-FLP/ (+ or Y ); FRT82B, Ubi-nGFP/FRT82B, Tctp h59 , hs-FLP/ (+ or Y ); FRT2A (=FRT79D-F), Ubi-nGFP/FRT2A, brm T362 . To generate Flip-out clones in SG, larvae were heat-shocked for 5 min at 38 °C at 24-48 h after egg deposit in the following genotypes: hs-FLP /(+ or Y ); UAS-Tctp-i/+; Ay-Gal4, UAS-GFP.S65T/+ hs-FLP /(+ or Y ); Ay-Gal4, UAS-GFP.S65T/UAS-Brm DN ::HA Eye pigmentation assay 2–3 days-old adult male flies were used for measuring eye pigmentation. Eye pigments were extracted from 20 frozen heads in 0.5 ml of cold acidified methanol (absolute MeOH with 0.1% HCl) using Kontes pestle. After centrifugation for 10 min at 12,000 r.p.m., 4 °C, the cleared lysate was collected into a new 1.5 ml tube. Absorbance at 480 nm was measured. Quantification was performed in triplicates. Quantitative real-time PCR Fly samples were frozen in liquid nitrogen and stored at –80 °C until use. Total RNA was prepared with Trizol reagent (Invitrogen, USA). Total RNA (2 μg) was reverse-transcribed using the QuantiTect reverse transcription Kit (Qiagen, Germany). Quantitative real-time PCR (QPCR) was performed using SYBR Green master mix on CFX96 Real-Time PCR System (Bio-Rad, USA) with standard cycling parameters (1 min at 95 °C and 40 cycles of 20 s at 95 °C, 20 s at 60 °C, and 45 s at 72 °C). C T values for the detected mRNA levels of each gene were normalized to those of rp49 . Mean expression levels were calculated from the values of three independent experiments, and were indicated as fold changes. Primer sets used for QPCR were listed in Supplementary Table 2 . Immunohistochemistry and western blotting SG and wing discs were fixed in PLP fixative (2% paraformaldehyde, 75 mM lysine, and 35 mM phosphate buffer, pH7.4) for 15–20 min at room temperature (RT). After brief washing two times in PBS for 10 min at RT, tissues were treated in blocking buffer (50 mM Tris-HCl, pH 6.8, 150 mM NaCl, 0.5% NP-40, and 5 mg per ml BSA) for 2 h at RT and incubated with primary antibody overnight at 4 °C in wash buffer (50 mM Tris-HCl, pH 6.8, 150 mM NaCl, 0.5% NP-40, and 1 mg per ml BSA). After washing four times in wash buffer for 40 min at RT, tissues were incubated with the appropriate secondary antibodies for 2 h at RT (1:300, Jackson immunoresearch). Primary antibodies were as follows: Mouse (Ms) anti-Fibrillarin (1:500, Abcam 4566), Rb (Rabbit) anti-H3K9me2 (1:200, Millipore 07-212), Rb anti-H3K9me3 (1:200, Abcam 8898), Ms anti-HP1a (1:50, DSHB C1A9-c), Rb anti-Tctp (1:1,000) [22] , [26] , Guinea Pig (GP) anti-Brm (1:400–500, y0866 from Dr. Fengwei Yu) [23] , FITC-Phalloidin (1:100, Sigma P5282), Rb anti-γ-H2Av (1:2,000, Rockland 600-401-914), Rat anti-HA (1:250, Roche 11867423). Chromosomes were visualized with DAPI. For confocal analysis, Zeiss LSM 710 was used. For polytene chromosome staining [67] , [68] , third instar larvae were raised at 18 °C to obtain well-resolved band/interband pattern. Primary antibodies were as follows: Rb anti-Tctp (1:300), Ms anti-HP1a (1:50, DSHB C1A9-c), GP anti-Brm (1:200), Ms anti-Pol-II (1:50, Covance MMS-128P), Ms anti-Pol-IIa (1:50, Covance MMS-126R), Ms anti-Pol-II Ser5 (1:50, Covance MMS-134R), and Ms anti-Pol-II Ser2 (1:50, Abcam 24758). Gross bands intensity on each channel was measured using ROI (Region of interest) menu in ZEN program (Zeiss) and normalized to DAPI intensity value using Excel program (Microsoft). For western blot analysis, 10 larvae or 20 pairs of third instar larval SG were lysed in SDS-gel leading buffer and analysed for each genotype. Primary antibodies were as follows: Rb anti-Tctp (1:20,000), Rb anti-Histone3 (1:10,000, Millipore 05-928), Ms anti-β-tubulin (1:5,000, DSHB E7-c), Ms anti-Fibrillarin (1:1,000, Abcam 4566), Ms anti-HP1a (1:1,000–2,000, DSHB C1A9-c), Ms anti-Pol-II (1:1,000, Abcam 5408), Ms anti-Pol-IIa (1:2,000, Abcam 817), Rb anti-Pol-II ser5 (1:2,000, Abcam 5131), and Rb anti-Pol-II Ser2 (1:2,000, Abcam 5095). Yeast two hybrid screen The full length Tctp bait (171 aa) was cloned into EcoRI/SalI sites of pGBKT vector as a EcoRI/XhoI fragment. Y2H Screening for Tctp partners was performed in yeast PBN204 strain containing three selection markers (URA3, lacZ and ADE2) that are under the control of different GAL promoters (PanBioNet, Pohang, Korea). Yeast transformants of the Tctp bait and Drosophila embryo cDNA AD library were spread on selection medium (SD-leucine, tryptophan, uracil (SD-LWU)) that supports growth of yeasts with bait and prey plasmids yielding proteins interacting each other. After selecting yeast colonies on uracil-deficient media, these URA + colonies were re-selected on adenosine-deficient media (SD-LWA). In vitro GST-pull down assay MBP-tagged Tctp [22] and GST-tagged Brm fragments (GST::Brm 1-311, 304-747, 748-1638, Δ304-500, Δ574-648, Δ694-747, ΔHSA, ΔBRK, and ΔHSA, ΔBRK) were cloned into pMAL-c2 (NEB) and pGEX5X-1 (GE healthcare), respectively. In-Fusion system (Clontech) was used for cloning. Primer sets used for cloning were listed in Supplementary Table 2 . GST-tagged and MBP-tagged proteins were expressed in E.coli Rosetta2 (Novagen, Germany). IPTG (0.1 mM) induction was performed in 14 °C shaking incubator at 250 r.p.m. for 4 h. The extracted proteins were dialysed in TBS buffer (10 mM Tris-HCl (pH8.0), 150 mM NaCl) containing 20% glycerol and 1 mM DTT and stored at -20 °C before use. Five micrograms of MBP fusion proteins were used as prey and the same amount of GST fusion proteins as baits. Protein complexes were formed in PDB (20 mM Tris-HCl (pH 7.5), 150 mM NaCl, 0.5 mM EDTA, 10% glycerol, 0.1% Triton X-100, 1 mM DTT, proteinase inhibitor cocktail (Roche)) containing 0.2% bovine serum albumin for 2–3 h at 4 °C. After washing three times in PDB at RT for 15 min, the samples were boiled in protein loading buffer at 94 °C for 5 min and loaded for western blotting. Primary antibodies were as follows: Ms anti-GST (1:4,000, SantaCruz sc-138) and Rb anti-MBP (1:10,000, NEB E8030S). Co-immunoprecipitation To express 2xFLAG-tagged full length Brm derivatives (WT, ΔHSA, ΔBRK, and ΔHSAΔBRK) in Drosophila S2 cell, PCR products amplified from LD36356 (DGRC, IN, USA) were cloned into pAc5.1-N’-tagged 2xFlag vector (modified from pAc5.1 (Invitrogen, USA)) using In-fusion system (Clontech). For C-terminus-V5-tagged ARP4 and Act expression, these genes were PCR-amplified from LD29458 and RE02927, respectively, and cloned into pAc5.1 vector. Primer sets used for cloning were listed in Supplementary Table 2 . 2xMYC-tagged Tctp is as reported previously [22] . For transfection, the amount of vector used per 1.2 × 10 6 cells were as follows: 0.25 μg of pAc5.1-2xMYC-Tctp, 0.5 μg of pAc5.1-2xFLAG-Brm (WT or derivatives), 0.5 μg of pAc5.1-ARP4-V5, and 0.5 μg of pAc5.1-Act-V5. S2 cells were transfected using X-tremeGENE HP DNA transfection reagent (Roche) according to the manufacturer’s manual with some minor modifications (3:1 ratio for transfection reagent per target DNA and 30 min incubation for transfection complex formation). pAc5.1 empty vector was used to transfect an equal amount of plasmids. Stable cell line expressing 2xFLAG-Brm WT were produced using pCoHygro (Invitrogen, 19:1=target:selection plasmids) and maintained in 10% AS (Sigma, I7267) containing M3 media with hygromycin B (Invitrogen, 10,687-010, 0.15 mg per ml). The nuclear extract was obtained from S2 cells and treated with 100 U per ml of benzonase (EMD Millipore) for 1 h in IP buffer (20 mM HEPES (pH 7.4), 0.2 mM EDTA, 1.5 mM MgCl2, 1 mM DTT, 5% glycerol, 80 mM KCl, 0.2% NP-40, 2 × proteinase inhibitor cocktail and 1x phostop (Roche)). Protein complexes were immunoprecipitated with each 5 microgram of Rb anti-MYC (Abcam 9106), Ms anti-FLAG (Sigma F1804), or Ms anti-Pol-II (Abcam 5408) at 4 °C for 2 h. The immunocomplexes were washed three times with cold IP buffer at 4 °C. The samples were boiled in protein loading buffer at 94 °C for 5 min and loaded for western blotting. Primary antibodies were as follows: Rb anti-FLAG (1:1,000, Cell Signaling #2368), Ms anti-MYC (1:2,000, SantaCruz, sc47694), Rb anti-MYC (1:10,000, Abcam 9106), Rb anti-V5 (1:2,500, Sigma v8137), and Ms anti-Pol-II (1:1,000, Abcam 5408). In vitro ATPase assay DNA-dependent ATPase activity was determined with a colorimetric assay measuring the formation of inorganic phosphate with some modifications [31] , [32] , [33] . Standard reaction mixtures (50 μl) contained 20 mM HEPES (pH 7.4), 0.2 mM EDTA, 1.5 mM MgCl 2 , 0.1 mM DTT, 5% glycerol, 80 mM KCl, 1 mM ATP, 20 μg ml −1 of SK(-) plasmid DNA, 2 × proteinase inhibitor cocktail (Roche). The reaction mixture was incubated at 30 °C for 30 min. Reaction was terminated by an addition of 0.85 ml of malachite green/acid molybdate/tween20 (0.04%) solution, followed by the addition of 0.1 ml of a 34% sodium citrate solution. After 15 min of color development, A660 was determined. Measuring eccDNA formation Approximately 100 larvae were frozen in liquid nitrogen. Samples were ground with a Kontes pestle in 0.5 ml of Hirt lysis buffer (0.6% SDS, 10 mM EDTA, pH 8.0) [6] , and then incubated at RT for 10–20 min. NaCl was added to a final 1 M concentration and incubated overnight at 4 °C. After centrifugation at 14,000 g for 40 min at 4 °C, the supernatant was collected into a new 1.5 ml tube and DNA was phenol-chloroform extracted three times and precipitated with ethanol. eccDNA content was assayed by QPCR and gel electrophoresis using appropriate primers ( Supplementary Table 2 ). Heat shock Third-instar larvae raised at 18 °C were transferred to 1.5 ml tubes containing a piece of wet 3MM paper and submerged in a 37 °C water bath for 30 min. Microarray analysis Total RNA was extracted using TRIzol reagent (Life Technologies, Carlsbad, CA, USA) according to the manufacturer’s protocol. Total RNA concentration and purity were determined by spectrophotometry to measure the absorbance ratio at 260:280 nm (RNA samples with ratios greater than 1.8 were used for analyses). The integrity of the RNA samples was also ascertained by analyzing 28S and 18S ribosomal RNAs with a Bioanalyzer 2100 (Agilent Technologies, Santa Clara, CA, USA). For gene expression profiles (eBiogen, Seoul, Korea), 500 ng RNA per sample was processed to labelled cRNA using the Affymetrix 3′ IVT Express kit according to the manufacturer's instructions and hybridized to Affymetrix Drosophila 2.0 GeneChips for 16 h at 45 °C. Gene chips were washed and stained with streptavidin-phycoerythrin using the Affymetrix Fluidics Station 450 and scanned on an Affymetrix GeneChip 3000 scanner (Affymetrix, Santa Clara, California, USA). The intensity values were normalized and summarized using robust multi-array analysis in R ( www.R-project.org ) and the Bioconductor package. A gene set representing >1.5-fold changes in at least one group ( Tctp h59/+ or Tctp EY/h59 ) is presented by hierarchical clustering analysis (red, >1.5-fold change; green, <1.5-fold change). The hierarchical clustering was conducted using Agilent's GeneSpring GX7.3 ( http://www.genomics.agilent.com/ ). Chromatin immunoprecipitation (ChIP) in S2 cells Cells (3.7–6.3 × 10 7 ) grown in a T25 flask were cross-linked with 1% formaldehyde for 10 min at room temperature. This cross-linking was stopped with 125 mM glycine for 5 min at room temperature. The DNA-protein complexes were prepared according to the manual for SimpleChIP enzymatic chromatin IP kit (Cell Signaling) without MNase treatment. The cross-linked chromatin was sheared into 200 ∼ 500 base pairs using Branson sonifier 450 (10% amplitude for 30 s with 0.5 s interval, five cycles). The DNA-protein complexes were incubated with each 2–3 μg of nonimmune IgG antibody, anti-PolII (Ab5408, 4H8), anti-H3 (Millipore 05-928), anti-H3K9me3 (Ab8898), anti-Brm (Dr Fengwei Yu) or anti-Tctp for overnight at 4 °C. Chromatin IP, bead-washing, and chromatin elution were performed according to the kit manual. Short DNA fragments corresponding to su(var)3-9 locus were amplified using QPCR. The primer set is listed in Supplementary Table 2 . Double-stranded RNA-mediated interference One microgram of PCR products with T7 promoter sequence ( pSK(-) or Tctp RNAi; Supplementary Table 2 ) was used for production of dsRNA (MEGAscript kit, Ambion). Bathing way was used for RNAi treatment. To maximize target protein reduction by Tctp RNAi, S2 cells were treated twice on day 0 and day 3 (or 4) [22] . Life span Flies were outcrossed 5 times with w 1118 to minimize genetic background effects. Life span was measured with 150–300 flies per genotype [69] . The life span of each genotype was measured at least in 8–15 separate vials (20 male flies a vial). Flies were cultured at 29 °C, 50% relative humidity, and 12:12 h light/dark cycle in an incubator. Food vials containing fresh standard corn-meal media were replaced every 2–3 days. Life span analyses was performed using PRISM 6 (GraphPad, USA) with the Kaplan–Meier method. Comparisons among groups were conducted using Log-rank test [70] . Data availability The microarray data are available at http://www.ncbi.nlm.nih.gov/geo/ (Accession number: GSE75900). All other relevant datasets will be made available from the authors upon request. How to cite this article: Hong, S.-T. & Choi, K.-W. Antagonistic roles of Drosophila Tctp and Brahma in chromatin remodelling and stabilizing repeated sequences. Nat. Commun. 7, 12988 doi: 10.1038/ncomms12988 (2016).